Bone remodelling in humans is load-driven but not lazy During bone remodelling, bone cells are thought to add and remove tissue at sites with high and low loading, respectively. To predict remodelling, it was proposed that bone is removed below and added above certain thresholds of tissue loading and within these thresholds, called a ‘lazy zone’, no net change in bone mass occurs. Animal experiments linking mechanical loading with changes in bone density or microstructure support load-adaptive bone remodelling, while in humans the evidence for this relationship at the micro-scale is still lacking. Using new high-resolution CT imaging techniques and computational methods, we quantify microstructural changes and physiological tissue loading in humans. Here, we show that bone remodelling sites in healthy postmenopausal women strongly correlate with tissue loading following a linear relationship without a ‘lazy zone’ providing unbiased evidence for load-driven remodelling in humans. This suggests that human and animal bones both react to loading induced remodelling in a similar fashion. A bone’s form follows its function—its shape, structure and mass are adapted to external forces acting on it. Already in the 19th century, a first indication for this functional adaptive phenomenon was given by suggesting that the internal structure of bones shows a similar orientation as principal stress trajectories [1] , [2] . It is thought that this form—function relationship is maintained by continuous remodelling of bone tissue where osteoblasts add bone at locations with high tissue loading and osteoclasts remove bone at locations with low tissue loading [3] . The relationship between bone remodelling and mechanical loading is usually assumed to follow the so-called Mechanostat Theory [4] . It states that bone mass is reduced below a lower threshold of mechanical tissue stimulus and increased above an upper threshold leading to a range where no net change occurs, called a ‘lazy zone’ or a ‘dead zone’ [5] , [6] , [7] , [8] , [9] , [10] . Many studies were conducted to figure out the response of bone to mechanical loading and thus to support the Mechanostat Theory. It was generally found that bone mass decreased in animals where hind limb bones were immobilized [11] , [12] or in participants of long-term bed rest studies [13] and astronauts [14] , [15] . On the other hand, bone mass increased when increased loading was applied to bone in vivo as shown in animal experiments, for example, in the turkey ulna [16] , mouse tibia [17] and mouse caudal vertebra [18] . Such an increased bone mass was also found in human, for example, in the playing arm of competitive tennis players [19] . Besides adapting its mass, bone can also adapt the orientation of its internal microstructure, which consists of a fine arrangement of small trabeculae, in response to changes in the orientation of loading. An experiment with juvenile guinea fowls showed that the trabecular orientation in the distal femur adjusted after altering the knee angles [20] . The same was later also demonstrated in the tarsal joint of juvenile sheep [21] . Due to the challenge of capturing bone microstructural changes in vivo , it was only recently that the load-adaptive behaviour of bone remodelling has been shown at the micro-scale in an animal study [22] . In vivo micro-computed tomography was used to study microstructural changes in mice caudal vertebra over time when applying non-physiological extra loading. By correlating the resulting sites of bone resorption and formation with local tissue loading as calculated with micro-finite element (micro-FE) analysis, a strong correlation between bone remodelling and local tissue loading was found while the results did not support the existence of a ‘lazy zone’. In spite of such evidence, people have questioned these experiments, arguing that skeletal changes could also have been evoked due to other causes than normal bone remodelling [23] . There are three reasons for these criticisms: first, surgery is required to apply controlled loading in vivo and this invasive procedure can lead to unpredictable osteogenic reactions. Second, experiments are usually done on juvenile animals that are still growing and thus growth processes confound any skeletal response. And third, the applied loading is often out of the physiological range to produce noticeable changes in bone mass. This could lead to fractures that trigger damage-repair processes that might involve reactions different from normal bone remodelling in the healthy state. To provide more convincing evidence for local load-adaptive regulation of bone tissue by bone cells, a strong correlation between bone remodelling sites and local mechanical loading at the bone micro-scale needs to be demonstrated without compromising the bone or its loading in any way, that is, for bone in its physiological state in vivo . Until recently, the analysis of bone microstructural changes and bone tissue loading in vivo was possible only in animal experiments [22] , but such studies could not exclude the confounding factors mentioned above. With the recent development of high-resolution imaging techniques; however, it has become possible to observe the bone microstructure and changes therein also for bone at human peripheral sites in vivo . In the present study, using such new imaging techniques allowing to assess microstructural changes in human bones in vivo , recently developed methods to quantify physiological tissue loading conditions, and data from healthy postmenopausal subjects to exclude growth, healing or other possibly confounding effects, we aim at verifying and quantifying the relationship between bone remodelling and mechanical loading at the micro-scale in humans. Therefore, we here investigate whether sites of bone resorption correlate with low tissue loading and sites of bone formation correlate with high tissue loading in healthy postmenopausal human bone under physiological conditions. Sites of bone remodelling are identified based on baseline and 2-year follow-up high-resolution peripheral quantitative computed tomography (HR-pQCT) images of the distal tibia of nine healthy postmenopausal women [24] , [25] , [26] . To calculate local tissue loading, micro-FE models are created from baseline and follow-up images, and a previously developed bone loading estimation algorithm [27] , [28] , [29] , [30] , [31] is used to determine the external loading history for each subject and measurement. Our study reveals, in human bone, a strong linear relationship between sites of bone remodelling and local tissue loading also influenced by non-mechanical remodelling events but not supporting the existence of a ‘lazy zone’. This is in agreement with recent animal studies [22] , [32] , suggesting that human and animal bones both react to loading induced remodelling in a similar fashion. Moreover, the agreement with the animal experimental results indicates that the absence of a ‘lazy zone’ is not the result of technical limitations when analysing human bone in vivo. The finding of a strong form—function relationship and its quantification further provides the basis for predicting bone remodelling in patients and for understanding bone microstructure. Finally, the proposed approach could be useful for defining the contribution of mechanical loading to the bone phenotype improving the knowledge of the development of bone shape during bone growth and evolution. Imaging and tissue loading HR-pQCT allows the assessment of the human distal tibia in vivo and in great detail ( Fig. 1a ). Registration of baseline and follow-up images reveals the sites of bone resorption and formation ( Fig. 1b ) and micro-FE calculations the tissue loading ( Fig. 1c ). 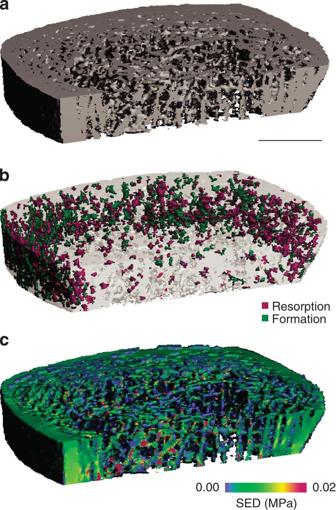Figure 1: Imaging and tissue loading. (a) Cross-section of the human distal tibia as assessed within vivoHR-pQCT, showing the region usually scanned in the clinics with a cut to reveal its internal microstructure. The length of the scale bar is 5 mm. (b) Sites of bone remodelling as determined using three-dimensional image registration of baseline and 2-year follow-up measurements. (c) Tissue loading represented as SED and calculated using micro-FE analysis. Figure 1: Imaging and tissue loading. ( a ) Cross-section of the human distal tibia as assessed with in vivo HR-pQCT, showing the region usually scanned in the clinics with a cut to reveal its internal microstructure. The length of the scale bar is 5 mm. ( b ) Sites of bone remodelling as determined using three-dimensional image registration of baseline and 2-year follow-up measurements. ( c ) Tissue loading represented as SED and calculated using micro-FE analysis. Full size image Correlating bone remodelling sites with tissue loading We find that bone resorption and formation are strongly correlated with local tissue loading and that bone resorption frequency peaks at low strain energy density (SED; average median=0.0088 MPa), whereas bone formation frequency peaks at high SED (average median=0.0141 MPa; Fig. 2a ). Subtracting resorption and formation histograms shows the quantitative relationship between bone remodelling and tissue loading. It indicates that there is a linear increase in bone remodelling within the physiological range of tissue loading and that the remodelling process is saturated at low and high tissue loading ( Fig. 2b ). 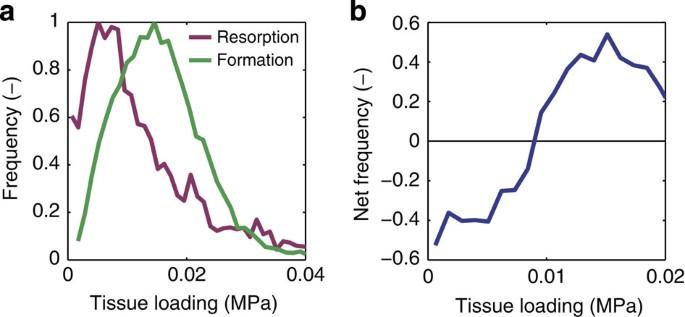Figure 2: Correlating bone remodelling sites with tissue loading. (a) Tissue SED histograms in the regions of bone resorption and formation. (b) Relationship between bone remodelling and tissue loading quantified by subtracting the formation and resorption histograms. Lines represent the average of all subjects (n=9). Figure 2: Correlating bone remodelling sites with tissue loading. ( a ) Tissue SED histograms in the regions of bone resorption and formation. ( b ) Relationship between bone remodelling and tissue loading quantified by subtracting the formation and resorption histograms. Lines represent the average of all subjects ( n =9). Full size image These results demonstrate a strong linear relationship between bone remodelling and local tissue loading providing evidence for bone’s load-adaptive behaviour at the micro-scale in humans. However, bone resorption and formation histograms also overlap considerably, indicating that bone remodelling is not purely load-driven. Possible causes for this could be that also other mechanisms, for example, calcium homeostasis, influence normal bone remodelling and thus bone is never fully load adapted. Calculating the coefficient of variation of the tissue loading gives us an impression of how much of the bone structure is determined by mechanical loading. For all nine subjects, we find a value of approximately 50%, which agrees with the indication that also other mechanisms influence bone remodelling and thus bone structure. It is thought that micro-cracks that occur at locations with high tissue loading induce bone resorption to replace old bone tissue [33] , [34] , [35] , [36] . Such resorption would correlate with high tissue loading and thus further explain the multifactorial nature of the relationship between bone remodelling and tissue loading. We earlier thought that part of this tissue loading inhomogeneity is due to bone’s unresponsiveness to mechanical loading within the ‘lazy zone’ [31] . However, we find a linear relationship between bone remodelling and tissue loading in the present study, which is not in agreement with a ‘lazy zone’. The existence of a ‘lazy zone’ was also investigated in recent animal experiments where loading was applied in vivo . In one study the osteogenic response was measured at different strain levels [32] and in another study bone remodelling probabilities were determined and correlated with tissue loading [22] ; however, in both cases no ‘lazy zone’ was found. Our study thus confirms these results for humans and indicates a combination of load-driven bone remodelling to adapt to external forces and non-mechanical remodelling events possibly to balance calcium levels and renew bone tissue. This combination would not lead to an equilibrium with a perfectly uniform tissue loading distribution and suggests that bone is only partially adapted to its external forces but is probably striving towards such a situation limited by the multifactorial nature of the remodelling process. There are also limitations to our study. First, the method to identify sites of bone remodelling might as well include differences between baseline and follow-up images that are not due to bone remodelling but due to movement artefacts of the scanning or registration inaccuracies. The high reproducibility of in vivo HR-pQCT [37] , however, indicates that microstructural changes can be identified well. And second, tissue loading is calculated based on an estimated loading history. Although the approach to determine subject-specific loading histories was validated earlier [27] and showed realistic results in human [28] , [29] , [30] , dog [28] and mouse [31] bone, it is only an estimate. We conclude that local tissue loading triggers sites of bone remodelling linearly dependent within a physiological range of tissue loading without a ‘lazy zone’ and that there is also a non-mechanical component in this relationship, possibly explained by remodelling activities fulfilling metabolic demands. Because the same relationship was also found in mouse bone, our results suggest that load-driven bone remodelling is similar in mice and humans. This supports the use of mouse models in bone research, particularly to investigate the influence of mechanical loading on bone remodelling. Moreover, the agreement with the animal experimental results indicates that the absence of a ‘lazy zone’ is not the result of technical limitations when scanning human bone in vivo (for example, the limited resolution and movement artefacts). By verifying and quantitatively describing the relationship between bone remodelling and tissue loading in humans, our study provides the fundamental basis for investigations for a variety of applications. These include predictions of bone remodelling around hip implants due to the reduction in loading conditions for bone near the implant (‘stress shielding’) [9] and clinical remodelling simulations to predict the development of diseases and to test different treatment options. Predictions of bone remodelling could also be used for tissue engineering, defining loading protocols that lead to tissue loading stimulating the cells as desired or for optimizing scaffold morphology and material properties. Our findings also provide convincing evidence for justifying form—function relationships in bone that are the basis for morphometric analyses of anthropological and palaeontological studies, for example, relating bone morphology to locomotor [38] or feeding [39] behaviour. Finally, our study concerns developmental biology as it helps revealing to what extent bone genotype and load adaptation determine the bone phenotype. Employing the presented approach in this research field could improve the knowledge of bone shape development during bone growth and evolution. Subjects and image acquisition High-resolution in vivo images of the distal tibia from a subset of healthy postmenopausal women ( n =9) with ages ranging from 59–80 years from the OFELY cohort [24] , [25] , [26] were used. Subjects were chosen randomly among measurements based on having no or minimal motion artefacts and thus high image quality. Baseline imaging started in 2005 and 2-year follow-up measurements continued in 2007. Subjects were assessed with HR-pQCT (XtremeCT, Scanco Medical AG, Switzerland) at an isotropic resolution of 82 μm at both, the distal radius and tibia, to assess the bone microstructure in a 9 mm cross-section. In addition, 15 healthy subjects with ages ranging from 21 to 47 years were assessed by three repeated in vivo scans at the distal radius and tibia within 1-month intervals [40] to investigate the short-term reproducibility. All subjects gave their informed consent and the local ethics committee (Comité Consultatif de Protection des Personnes dans la Recherche Biomédicale de Lyon A) approved the study. Bone remodelling sites quantification To identify locations of bone resorption and formation, follow-up images were registered to baseline images using rigid three-dimensional registration and voxels at the bone surface were categorized either into a resorption site, a formation site, or an unchanged site ( Fig. 1b ). It was recently investigated that the presented three-dimensional registration method provides accurate results based on in vivo HR-pQCT images [37] . Individual voxel densities of the common region of the registered images were subtracted voxel by voxel and a change in density below or above 225 mg HA per ccm was defined as resorption and formation, respectively. To remove noise, only changes leading to a cluster of a minimum of 30 voxels were included. The threshold and cluster size parameters were chosen based on running the image analysis on the in vivo short-term reproducibility dataset in such a way that the resorption and formation were below 2.5% of the total number of bone voxels at baseline, which is consistent with the reproducibility of in vivo HR-pQCT [37] . The image-processing algorithm was implemented using Image Processing Language (IPL, Scanco Medical AG). Tissue loading calculation Micro-FE models were created from baseline and follow-up images for all subjects by transforming each voxel into an equally sized brick-element with a resolution of 82 μm (IPLFE, Scanco Medical AG). Earlier mesh convergence studies suggest that the image resolution of 82 μm is still adequate for accurate finite element analyses in general [41] , [42] , [43] , while the element size over structural length ratio (0.009) in the present study is still within a well acceptable range [44] . Subject-specific loading conditions were determined using a previously developed and validated bone loading estimation algorithm [27] , [28] , [29] , [30] , [31] . Specifically to the bone loading estimation algorithm, we found that calculated normal forces in cubic bone microstructures differ by less than 20% when changing the resolution from 20 to 80 μm, indicating little image resolution dependency in that range [28] . Although discretization and other errors in the solution could affect the SED calculation, the fact that we found a clear correlation between the local SED magnitude and bone remodelling indicates that such errors are likely small and do not affect our conclusions. Bone was modelled as homogenous linear elastic material with a Young’s modulus of 6.8 GPa and a Poisson’s ratio of 0.3. In earlier validation studies, it was found that these material properties provide good agreement between experimentally measured and calculated stiffness of scanned bone segments in a uniaxial compression test [45] . Incorporating the bone microstructure into the model accounts for the anisotropy of trabecular bone structure and thus allows using such simple material properties [45] . To achieve a realistic load transfer as well as to distribute the applied loading, a layer of soft material with a Young’s modulus of 15 MPa was added at both ends of the models [29] . The models were then used to calculate the actual tissue loading ( Fig. 1c ). Using the estimated bone loading as boundary conditions for the micro-FE models, the tissue loading, represented as SED values, were calculated and averaged between baseline and follow-up images. Averaging SED values required overlapping regions between baseline and follow-up images, which was achieved by dilating resorption and formation sites by one voxel. Only averaged SED values within the common region of baseline and follow-up images corresponding to dilated resorption or formation sites were used, ensuring that all resorption and formation voxels have a corresponding averaged SED value. Results representation SED frequency distributions were calculated for bone resorption and formation voxels separately and represented in histograms ( Fig. 2 ). Since the total amount of bone resorption and formation can differ substantially between subjects, making it difficult to compare the resulting frequency curves, the histograms were normalized with respect to the total number of resorption and formation voxels, respectively. How to cite this article: Christen, P. et al. Bone remodelling in humans is load-driven but not lazy. Nat. Commun. 5:4855 doi: 10.1038/ncomms5855 (2014).